Mudskipper genomes provide insights into the terrestrial adaptation of amphibious fishes Mudskippers are amphibious fishes that have developed morphological and physiological adaptations to match their unique lifestyles. Here we perform whole-genome sequencing of four representative mudskippers to elucidate the molecular mechanisms underlying these adaptations. We discover an expansion of innate immune system genes in the mudskippers that may provide defence against terrestrial pathogens. Several genes of the ammonia excretion pathway in the gills have experienced positive selection, suggesting their important roles in mudskippers’ tolerance to environmental ammonia. Some vision-related genes are differentially lost or mutated, illustrating genomic changes associated with aerial vision. Transcriptomic analyses of mudskippers exposed to air highlight regulatory pathways that are up- or down-regulated in response to hypoxia. The present study provides a valuable resource for understanding the molecular mechanisms underlying water-to-land transition of vertebrates. The water-to-land transition during the Devonian period is one of the most significant events in the evolutionary history of vertebrates and led to the emergence of tetrapods, the most successful group of animals on land. Interestingly, several groups of teleosts that emerged much later in evolution have independently evolved adaptations that enable them to spend a considerable part of their life on land. These terrestrial adaptations include aerial respiration, higher ammonia tolerance, modification of aerial vision and terrestrial locomotion using modified pectoral fins. However, very little is known about the genetic basis of these adaptations. Mudskippers (family Gobiidae; subfamily Oxudercinae) are the largest group of amphibious teleost fishes that are uniquely adapted to live on mudflats. They include four main genera, namely, Boleophthalmus , Periophthalmodon , Periophthalmus and Scartelaos [1] comprising diverse species that represent a continuum of adaptations towards terrestrial life with some being more terrestrial than the others. Thus, mudskippers are a useful group for gaining insights into the genetic changes underlying the terrestrial adaptations of amphibious fishes. Here we report whole-genome sequencing of four representative species of mudskippers: B. pectinirostris (BP or blue-spotted mudskipper), S. histophorus (SH or blue mudskipper), Periophthalmodon schlosseri (PS or giant mudskipper) and Periophthalmus magnuspinnatus (PM or giant-fin mudskipper). BP and SH are predominantly aquatic and spend less time out of water whereas PS and PM are primarily terrestrial and spend extended periods of time on land ( Fig. 1 ). Comparative analyses are carried out to provide insights into the genetic basis of terrestrial adaptation in mudskippers. 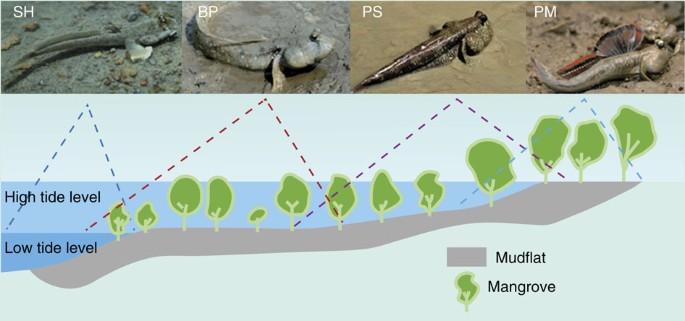Figure 1: Habitats of the four sequenced mudskippers. BP and SH are predominantly water dwelling, whereas PM and PS spend extended periods of time on land. Interestingly, the genome size decreases in the following order: BP>SH>PS>PM, which may be associated with their terrestrial affinity but unrelated to their body size (PS>BP>SH>PM). Figure 1: Habitats of the four sequenced mudskippers. BP and SH are predominantly water dwelling, whereas PM and PS spend extended periods of time on land. Interestingly, the genome size decreases in the following order: BP>SH>PS>PM, which may be associated with their terrestrial affinity but unrelated to their body size (PS>BP>SH>PM). Full size image Assembly and annotation A series of sequencing libraries were constructed from genomic DNA of the four mudskippers. In total, 232.72, 93.80, 79.74 and 66.65 gigabases (Gb) of raw data were generated using the Illumina HiSeq 2000 platform for BP, PM, SH and PS, respectively ( Supplementary Note 1 and Supplementary Table 1 ). The SOAP denovo 2 (ref. 2 ) assembled genome sizes of these four mudskippers are 0.966, 0.715, 0.720 and 0.683 Gb, respectively. 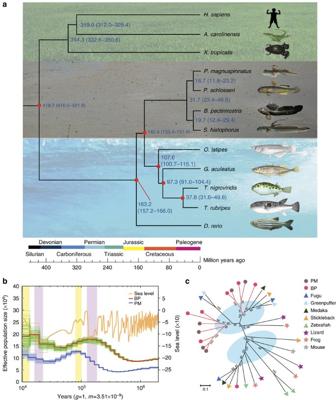Figure 2: The phylogenetic placement, demographic history and specific TLR13 expansion of mudskippers. (a) A phylogenetic tree was constructed using fourfold degenerate sites of 1,913 genes from 12 vertebrate species. Blue numbers at the nodes represent divergence time between lineages. Red dots indicate the reference divergence times from the TimeTree (http://www.timetree.org/). (b) The population history of two representative mudskippers (BP and PM) was estimated. The red and blue lines represent the population size changes in BP and PM, respectively. The green and light blue lines, around the red and blue lines, are the PSMC estimates on 100 sequences randomly re-sampled from the original sequences. The orange line denotes the fluctuation of the global sea level. (c) Phylogeny of TLR13 family in ten representative vertebrates showing the expansion of TLR13 in mudskippers. The details of their contig N50 and scaffold N50 values are provided in Table 1 and Supplementary Table 2 . The quality of the genome assemblies was evaluated using five different criteria ( Supplementary Note 1 ). Our assessment confirms that the BP genome assembly is of high quality and can be used as the reference mudskipper genome. In addition, the PM genome assembly has long contigs (N50 of 27.6 kb) and can be useful for genome-wide comparisons with BP. Besides BP and PM genomes, we also annotated protein-coding genes in the ‘draft’ assemblies of SH and PS genomes and used them to determine phylogenetic relationships of the four sequenced mudskippers ( Fig. 2a ). We employed a standard annotation pipeline to predict gene sets of the four mudskippers, resulting in 20,798, 20,927, 18,156 and 17,273 genes in BP, PM, SH and PS, respectively ( Supplementary Note 2 and Supplementary Figs 6 and 7 ). BP has the highest concentration of transposable elements (TEs) and a remarkable expansion of the hAT superfamily, which may explain its largest genome size among the four species ( Supplementary Table 7 ). Table 1 Genome sizes and assembly statistics of the four mudskipper genomes. Full size table Figure 2: The phylogenetic placement, demographic history and specific TLR13 expansion of mudskippers. ( a ) A phylogenetic tree was constructed using fourfold degenerate sites of 1,913 genes from 12 vertebrate species. Blue numbers at the nodes represent divergence time between lineages. Red dots indicate the reference divergence times from the TimeTree ( http://www.timetree.org/ ). ( b ) The population history of two representative mudskippers (BP and PM) was estimated. The red and blue lines represent the population size changes in BP and PM, respectively. The green and light blue lines, around the red and blue lines, are the PSMC estimates on 100 sequences randomly re-sampled from the original sequences. The orange line denotes the fluctuation of the global sea level. ( c ) Phylogeny of TLR13 family in ten representative vertebrates showing the expansion of TLR13 in mudskippers. Full size image Population history We identified 1,683,572 and 820,179 heterozygous single-nucleotide variations in the BP and PM genomes, respectively. The corresponding heterozygosity rates are 0.188% and 0.117%. The demographic history of BP and PM from 2,000,000 to 10,000 years ago (Pleistocene) was reconstructed with these heterozygous SNVs using the Pairwise Sequentially Markovian Coalescent (PSMC) model [3] ( Fig. 2b ). The population size of BP was estimated to be always larger than that of PM. The demographic expansion or bottleneck events in their population history showed a remarkable relation to the eustatic sea-level fluctuations. The largest population sizes of BP occurred when the sea was at a lower level whereas PM population sizes were the largest when the sea was at a higher level. These observations could be related to differences in habitat and food availability as the sea level fluctuated. BP prefers mudflats [4] and mainly feeds on benthic diatoms [1] , which are particularly abundant on intertidal mud deposits; PM, on the other hand, is an opportunistic carnivore [1] and prefers grass-dominated, mid-high intertidal marshes [5] . Therefore, low sea level could have offered more mudflats to grow diatoms for the propagation of BP. Conversely, high sea level would have provided wider marsh habitats for PM to catch insects and crustaceans [1] and hence to generate a large population. Reinterpretation of mudskipper phylogeny We determined the phylogenetic relationships and divergence times of the four mudskippers and eight representative vertebrates using 1,913 single-copy orthologous genes ( Fig. 2a ). The phylogenetic tree clearly shows that the four mudskippers form a monophyletic clade which diverged from the other teleosts ~140 Myr ago. Within this clade, SH and BP form one sister group, whereas PS and PM constitute another sister group, which is consistent with the former two being predominantly aquatic and the latter two being more terrestrial. This topology is in contrast to the morphology-based cladistic tree proposed by Murdy [6] ( Supplementary Fig. 12 ), which suggested that SH was an outgroup to a clade comprising BP, PS and PM. We confirmed our inferred phylogeny by using different data sets and three different standard phylogenetic methods ( Supplementary Fig. 13 ). Immune and DNA metabolism adaptation on land After diverging from other teleosts, mudskippers have acquired many genes that are crucial for existence in their unique ecological niches. To investigate this aspect of the water-to-land transition, we identified 684 genes (657 genes possess transcript evidence; see Supplementary Note 5 ) that are present in mudskippers but not in other analyzed teleosts. These genes are significantly enriched (false discovery rate <0.001) in immune domains such as ‘Immunoglobulin-like’, ‘Immunoglobulin V-set’ and ‘Immunoglobulin subtype’. In particular, they include four complete genes for the toll-like receptor 13 (TLR13), a family of innate immune receptors that can recognize 23S rRNA in bacteria [7] . In fact, the mudskippers possess the largest number (11 copies) of TLR13 in sequenced vertebrates so far ( Supplementary Table 13 ). Phylogenetic analysis showed that the vertebrate TLR13 forms two distinct clades representing two subfamilies ( Fig. 2c ), and that only one of the subfamilies has expanded in mudskippers. Gene duplication could facilitate adaptation by neofunctionalization [8] . These gained TLR13 and other immune-domain-containing genes may provide special immune defence against novel pathogens encountered on land. This hypothesis needs to be verified by analyzing the genome of a non-amphibious goby and determining whether the expansion of these gene families has occurred specifically in amphibious mudskippers. Strong terrestrial adaptations of mudskippers are likely to be the result of intense selective pressure acting independently on different gene families. We identified 722 and 705 positively selected genes (PSGs) in the BP and PM lineages from 4,844 one-to-one orthologues in the two mudskippers and five representative teleost genomes ( Supplementary Note 5 ). These mudskipper PSGs are markedly enriched in the gene ontology terms ‘DNA repair’, ‘DNA replication’, ‘nucleic acid metabolic process’ and ‘response to stress’ ( Supplementary Fig. 15 and Data 2 ), which is consistent with their roles in maintaining genomic stability and responding to the harsh temperature gradients and direct sunlight [9] in the intertidal zone. Ammonia excretion in the gill Mudskippers have a greater capacity to detoxify ammonia than many other aquatic species. However, they do not make use of the ornithine–urea cycle to produce urea as a means of detoxifying ammonia like tetrapods [10] . Their remarkably high tolerance to environmental ammonia and ability to survive on land are related to a combination of active NH 3 /NH 4 + excretion and low membrane permeability for ammonia [11] . To understand the selective pressure operating on the ammonia excretion pathway, we examined nine key genes that encode core proteins of the ammonia excretion pathway in the gill ( Fig. 3a ). Interestingly, carbonic anhydrase 15 and Na + /H + exchanger 3 in BP, and carbonic anhydrase 15 and glycosylated Rhesus protein c 1 (Rhcg1) in PM were found to be under significant positive selection ( Supplementary Table 14 ). Carbonic anhydrase catalyzes the reversible reaction: CO 2 +H 2 O←HCO 3 − +H + , which supplies protons for trapping NH 4 + both in the cytoplasm and gill boundary-layer water [12] . Na + /H + exchanger is involved in regulating Na + /NH 4 + exchange [13] and Rhcg1 controls nonionic NH 3 transport [14] . Positive selection of these genes suggests a role for them in the more-efficient ammonia excretion in the gills of mudskippers. 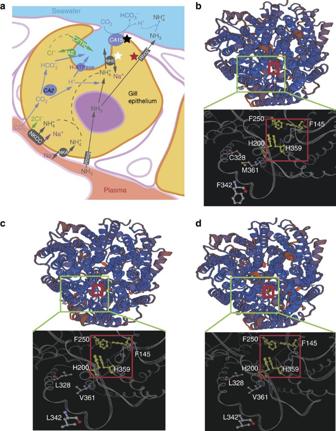Figure 3: Differential ammonia excretion in the gills of mudskippers. (a) An overview of ammonia excretion pathways in the gills illustrates the differential ammonia excretion in mudskippers. The core pathway comprises Na+–K+–Cl−co-transporter (NKCC), Na+K+–ATPase (NKA), carbonic anhydrase (CA), cystic fibrosis transmembrane conductance regulator (CFTR), Na+/H+exchanger (NHE) 3, H+–ATPase-V-type-B-subunit (H–ATPase), anion exchanger (AE), glycosylated Rhesus protein b (Rhbg) and c (Rhcg1 and Rhcg2). The black star represents genes with positive selection in both BP and PM, whereas the white and red stars indicate genes that are positively selected specifically in BP and PM, respectively. (b–d) Three-dimensional views of Rhcg1 proteins in BP (b), PM (c) and PS (d) highlight several PM- and PS-specific amino-acid substitutions. The red squares indicate the central pore of the channel for transporting NH3, which includes the conserved Phe-Gate (F145, F250) and Twin-His (H200, H359). Three genetic variations around the central pore, Leu328Cys, Leu342Phe and Val361Met in PM and PS, may be related to a more-efficient NH3diffusion system in PM and PS suited for a land-dominant lifestyle. Figure 3: Differential ammonia excretion in the gills of mudskippers. ( a ) An overview of ammonia excretion pathways in the gills illustrates the differential ammonia excretion in mudskippers. The core pathway comprises Na + –K + –Cl − co-transporter (NKCC), Na + K + –ATPase (NKA), carbonic anhydrase (CA), cystic fibrosis transmembrane conductance regulator (CFTR), Na + /H + exchanger (NHE) 3, H + –ATPase-V-type-B-subunit (H–ATPase), anion exchanger (AE), glycosylated Rhesus protein b (Rhbg) and c (Rhcg1 and Rhcg2). The black star represents genes with positive selection in both BP and PM, whereas the white and red stars indicate genes that are positively selected specifically in BP and PM, respectively. ( b – d ) Three-dimensional views of Rhcg1 proteins in BP ( b ), PM ( c ) and PS ( d ) highlight several PM- and PS-specific amino-acid substitutions. The red squares indicate the central pore of the channel for transporting NH 3 , which includes the conserved Phe-Gate (F145, F250) and Twin-His (H200, H359). Three genetic variations around the central pore, Leu328Cys, Leu342Phe and Val361Met in PM and PS, may be related to a more-efficient NH 3 diffusion system in PM and PS suited for a land-dominant lifestyle. Full size image Since amino-acid substitutions can affect the physicochemical properties of the Rhcg protein thereby affecting NH 3 permeation [15] , we examined the predicted three-dimensional structures of Rhcg1 in BP and PM based on information from the human RhCG [16] . Three genetic variations around the central pore of the channel for transporting NH 3 were identified between PM and BP (Leu328Cys, Leu342Phe and Val361Met) ( Fig. 3b,c ), resulting in more hydrophobic residues lining the central pore in PM. These residues should enhance the passage of NH 3 through the Rhcg1 channel, implying that Rhcg1 may be more effective for NH 3 transport in PM than BP. Similarly, Rhcg1 of PS is also under significant positive selection and shares several specific amino-acid changes with Rhcg1 of PM ( Fig. 3d and Supplementary Fig. 16 ). This might provide a molecular explanation for the previous finding [17] that the predominantly terrestrial species PS excreted more ammonia to the external medium than the largely aquatic species B. boddaerti when they were exposed to seawater containing 8 m M NH 4 Cl ( Supplementary Table 15 ). Vision modification Fully aquatic teleost fishes are likely to have myopic vision in air. However, mudskippers seem to have good aerial vision as evident from their ability to avoid terrestrial predators [18] . Comparison of vision-related genes in the two representative mudskippers (BP and PM) and several representative vertebrates highlighted certain vision-related genes that have been adaptively lost or mutated in mudskippers. Visual pigments consist of an opsin and a chromophore which are covalently joined via a Schiff’s base. Five visual opsin gene subfamilies, including LWS (long wavelength-sensitive), SWS1 (short wavelength-sensitive 1), SWS2 (short wavelength-sensitive 2), RH1 (rhodopsin) and RH2 (green-sensitive), have been reported in the vertebrate retina. From our genome data, we identified only four opsin subfamilies in BP and PM, and found that both mudskippers have lost SWS1 ( Supplementary Fig. 19 ). This loss of SWS1 could be a consequence of increased exposure of mudskippers to ultraviolet light during their forays out of water. SWS1 is often used for ultraviolet vision. Since ultraviolet can be damaging to the retina [19] , many vertebrates (i.e., human, cow, chicken, etc. ), have developed protective mechanisms to minimize retinal damage from ultraviolet and their SWS1s have shifted more towards violet rather than ultraviolet [20] . Mudskippers may have overcome this problem by making SWS1 less effective, and allowing it to be lost from the genome. We estimated the peak absorption spectra ( λ max , Table 2 ) of LWS of mudskippers based on five crucial sites (S180A, H197Y, Y277F, T285A and A308S) [21] . Our data show that the two mudskippers have a broader range of colour sensitivities between LWS1 and LWS2 than other teleosts. In fact, the sensitivity range of BP is comparable to that of human. Therefore, it seems that the two LWS opsins in mudskippers are adapted for aerial vision and for enhancement of colour vision. Table 2 Maximal absorption spectrum ( λ max ) of long wavelength-sensitive opsins (LWS). Full size table Arylalkylamine N -acetyltransferase (AANAT) is the most crucial enzyme that drives the large daily cycles of melatonin biosynthesis. A single AANAT gene is present in tetrapods (mammals, birds, reptiles and amphibians), whereas teleosts possess two copies of AANAT1 (AANAT1a and AANAT1b) and one copy of AANAT2. We noted that BP contains all three AANATs whereas PM possesses only AANAT1b and AANAT2. The loss of AANAT1a from the PM genome was confirmed by the lack of PM reads mapping to the AANAT1a sequence of BP ( Supplementary Fig. 17 ). Dopamine acetylation is a novel function of AANAT1a in the retina [22] and has been proposed to cause low retinal-dopamine levels leading to myopia development [23] . We speculate that the loss of AANAT1a in PM may lead to a reduction in the occurrence of myopia (through higher retinal-dopamine levels) which would facilitate aerial vision, a selective advantage for PM which spends most (over two-third) of its lifetime on the mudflat surface. However, further comparative studies of retinal-dopamine levels and aerial visual capabilities of PM and BP need to be carried out to verify this possibility. Shift in olfactory and vomeronasal receptor gene repertoire Olfaction is vital for finding food and mates and also for avoiding predators. Odorant molecules present in the environment are perceived through olfactory receptors. We characterized olfactory receptor (OR) genes and identified 32 and 33 OR-like genes in the BP and PM genomes, respectively ( Supplementary Table 16 ). Based on the nomenclature of Niimura [24] , 20 genes of BP and 17 genes of PM fall under the ‘delta’ class of ORs ( Supplementary Table 16 ), which are involved in the perception of water-borne odorants. Given that other teleost fishes contain 30–71 delta class ORs (see Supplementary Table 16 and Supplementary Fig. 22 ), mudskippers have experienced a contraction of this group of ORs. This suggests that mudskippers have limited perception of water-borne odorants compared with other teleosts. Intriguingly, neither mudskipper contains ORs belonging to the alpha or gamma group, which are required for air-borne odorant perception. On the contrary, most land vertebrates contain up to 200 and 1,200 members of alpha and gamma group ORs, respectively [24] . The absence of these genes in mudskippers is surprising, given the fact that they spend considerable amount of time on land for feeding and courtship. Besides the main olfactory system, many vertebrates also possess an accessory olfactory system known as the vomeronasal system which is involved in detection of intraspecific pheromonal cues and some environmental odorants. There are two categories of vomeronasal receptors called V1R and V2R. V1Rs bind to small air-borne chemicals, whereas V2Rs bind to water-soluble molecules [25] , [26] . Typical terrestrial vertebrates contain more V1R genes than V2R genes, and most teleost fishes contain more V2R than V1R genes ( Supplementary Table 17 ). We found that mudskippers contain more V1Rs and fewer V2Rs than other teleost fishes ( Supplementary Table 17 and Supplementary Fig. 23 ). It is therefore possible that mudskippers might be using V1Rs for detecting air-borne chemicals on land like tetrapods. Desiccation and hypoxia adaptive responses Terrestrial life exposes mudskippers to desiccation and hypoxia for most of their lifetime. To understand how mudskippers adapt to these altered environments, we analyzed gene expression patterns in multiple tissues (brain, skin, liver, muscle and gill) of BP and PM during a 6-h air-exposure experiment (samples collected at 0, 3 and 6 h; Supplementary Note 6 ). We identified 5,651 and 5,222 genes (from BP and PM) that were significantly up- or down-regulated in at least one tissue ( Supplementary Figs 24,25 and Table 18 ). Our transcriptome analysis uncovered a comprehensive set of genes downregulated in all the five tissues of BP and PM. These genes are significantly enriched ( P value<0.001, fold change ≧ 2) in ‘focal adhesion’, ‘ECM-receptor interaction’ and ‘Cytokine-cytokine receptor interaction’ pathways of the KEGG ( Supplementary Fig. 26 and Table 19 ). The downregulation of genes in these pathways is known to result in the inhibition of cell migration, stress fibre contraction and proliferation [27] , [28] , [29] , [30] . These results are consistent with previous findings based on hypoxia experiments in zebrafish [31] and medaka [32] , which suggested that fishes employ an energy-saving strategy associated with suppression of cell-growth and proliferation under hypoxic conditions. In addition, expression of the transforming growth factor-beta (TGF-beta) family members and genes related to blood cell development were also remarkably suppressed in mudskippers ( Supplementary Table 19 ). Among the upregulated genes, ( Supplementary Table 20 ) fructose- and mannose-metabolism pathway genes were significantly enriched in the liver ( P value<0.001, fold change ≧ 2), indicating a potential shift towards anaerobic ATP production under hypoxia and desiccation [33] . Conclusion Amphibious fishes such as mudskippers are an interesting group of vertebrates that can thrive in water as well as on land. They evolved independently and more recently than the lobe-finned fishes that made a successful transition from aquatic life to terrestrial living around 360 Myr ago resulting in the evolution of terrestrial tetrapods. Since the intermediary forms that existed during the transition from aquatic lobe-finned fishes to terrestrial tetrapods are represented currently only in fossils, amphibious fishes offer a useful model for understanding genetic changes associated with the water-to-land transition of vertebrates. Our analysis of four mudskipper genomes has provided insights into a variety of genetic changes that are likely associated with land adaptation of these amphibious fishes. Further experiments are required to establish cause-and-effect relationships between these genetic changes and the adaptations of mudskippers. The genomic and transcriptomic data developed in this study provide a useful resource for such studies. Genome sequencing and assembly Wild individuals of BP (female, 1 year old), PM (female, 1 year old) and SH (female, 1 year old) were collected from Shenzhen Bay at Shenzhen and Qiao Island at Zhuhai, Guangdong Province, China in July of 2012 and PS (female, 1 year old) samples were collected in Malaysia. All animal experiments in this study were performed in accordance with the guidelines of the animal ethics committee and were approved by the Institutional Review Board on Bioethics and Biosafety of BGI. Genomic DNA was isolated from several mixed tissues by standard molecular biology techniques. Whole-genome shotgun-sequencing strategy was employed and subsequent short-insert libraries (170-bp, 250-bp, 500-bp and 800-bp for BP; 250-bp and 800-bp for PM and SH; 170-bp, 500-bp and 800-bp for PS) and long-insert libraries (2-kb, 5-kb, 10-kb and 20-kb for BP; 2-kb for PM) were constructed using the standard protocol provided by Illumina (San Diego, USA). Paired-end sequencing was performed using the Illumina HiSeq 2000 system. In total, we obtained 232.72, 93.80, 79.74 and 66.65 Gb ( Supplementary Table 1 ) of raw reads from the libraries of BP, PM, SH and PS, respectively. SOAP denovo2 ( http://soap.genomics.org.cn/ , version 2.04.4) [2] with optimized parameters (pregraph -K 27 -p 16 -d 1; contig –M 3; scaff -F -b 1.5 -p 16) was used to construct contigs and original scaffolds. All reads were mapped onto the contigs for scaffold building by utilizing the paired-end information. This paired-end information was subsequently applied to link contigs into scaffolds in a stepwise manner. Some intra-scaffold gaps were filled by local assembly using the reads in a read-pair where one end was uniquely mapped to a contig whereas the other end was located within a gap. Subsequently, SSPACE [35] (version 2.0; using core parameters ‘-k 6 -T 4 -g 2’) was used to link the SOAP denovo2 scaffolds of BP and PM into super scaffolds with large-insert reads (>1 kb). Repetitive sequence detection and gene prediction We constructed a de novo repeat library using RepeatModeller (default parameter) and LTR_FINDER [36] . To identify known and de novo TEs, we employed RepeatMasker [37] ( http://www.repeatmasker.org/ , version 3.2.9) against the Repbase [38] TE library (version 14.04) and the de novo repeat library. In addition, we used RepeatProteinMask (version 3.2.2) implemented in RepeatMasker to detect the TE-relevant proteins. We also predicted tandem repeats utilizing Tandem Repeat Finder [39] (version 4.04) with parameters set as ‘Match=2, Mismatch=7, Delta=7, PM=80, PI=10, Minscore=50, and MaxPerid=2000’. Protein-coding gene annotation was combined by three parts: (1) Homology-based gene prediction: we aligned H. sapiens (human), D. rerio (zebrafish), T. rubripes (fugu), T. nigroviridis (greenpuffer), G. aculeatus (stickleback) and O. latipes (medaka) proteins (Ensembl release 64) to the BP and PM genomes using TblastN with E value≤1E-5, and then made use of Genewise2.2.0 (ref. 40 ) for precise spliced aligning and predicting gene structures. (2) Ab initio prediction: genome sequences of BP and PM were repeat-masked and 1,500 full-length and random-selected genes from their homology gene sets were used to train the model parameters for AUGUSTUS. Subsequently, we utilized AUGUSTUS2.5 (ref. 41 ) and GENSCAN1.0 (ref. 42 ) for de novo prediction on repeat-masked genome sequences. Short genes were discarded using the same filter threshold as for homology prediction. (3) Transcriptome gene prediction: we mapped the mixed RNA reads from liver, muscle, skin, gill and brain samples (details of RNA sample preparation are given in Supplementary Note 3 ) of BP and PM to their genomes respectively using Tophat1.2 (ref. 43 ). Subsequently, we sorted and merged the Tophat mapping results and then applied Cufflink ( http://cufflinks.cbcb.umd.edu/ ) [44] software to identify gene structures to assist gene annotation. Finally, all the above gene sets were merged to form a comprehensive and non-redundant gene set using GLEAN [45] ( Supplementary Fig. 6 ). Air-exposure experiment Six individuals, each measuring ~5 cm, were placed in Tris (pH 7.0)—15‰ artificial seawater as controls. Ten individuals were placed in plastic aquaria without seawater for air-exposure; the room temperature and humidity were maintained at 27±0.5 °C and 75±3%, respectively. Samples from the controls were collected at time point zero, whereas tissues were collected at 3 and 6 h after the air-exposure treatment. For the collection of samples, each fish was killed with a single blow on its head. The gill, brain, liver, skin and muscle were collected immediately. No attempt was made to separate the red and white muscle. The samples were immediately freeze-clamped in liquid nitrogen with pre-cooled aluminium tongs. All samples were stored at −80 °C until use. The details of expression calculation and differentially expressed gene detection were shown in Supplementary Note 3 . Estimation of demographic fluctuations using PSMC The distribution of time to TMRCA (the most recent common ancestor) between two alleles in an individual can be related to the history of population size fluctuation. To estimate the demographic TMRCA history of BP and PM, we performed the PSMC model [3] on heterozygous sites of BP and PM genomes ( Supplementary Note 4 ) with the generation time (g=1 year) [46] and the mutation rate (μ=3.51 × 10 −9 per year per nucleotide) [47] . Finally, we used gnuplot4.4 (ref. 48 ) to draw the reconstructed population history ( Fig. 2b ). Evolutionary analysis (1) Gene family construction: reference protein sequences of H. sapiens (human), D. rerio (zebrafish), T. rubripes (fugu), X. tropicalis (African frog), G. aculeatus (stickleback), T. nigroviridis (greenpuffer), A. carolinensis (lizard) and O. latipes (medaka) were downloaded from the Ensembl Core database (release 64). The consensus proteome set of the above eight species and our four mudskippers were filtered to remove those protein sequences <50 amino acids and resulted in a data set of 239,304 protein sequences that was submitted to OrthoMCL [49] for protein clustering. A total of 21,149 OrthoMCL groups were built utilizing an effective database size of 239,304 sequences for all-to-all BLASTP strategy with an E value=1E-5 and a Markov Chain Clustering (MCL) default inflation parameter. (2) Building the phylogenetic tree: we extracted 1,913 single-copy (only one gene from each species) families from 12 vertebrate species. Multiple alignments were performed on proteins of each selected family by MUSCLE (version 3.8.31) (ref. 50 ) and we converted protein alignments to their corresponding CDS alignments using an in-house perl script. All the translated CDS sequences were combined into one ‘supergene’ for each species. Fourfold degenerate sites (4D) extracted from the supergenes were then joined into new 4D genes of every species to construct a phylogenetic tree using MrBayes Version 3.2 (ref. 51 ) (GTR+gamma model). (3) Estimating divergence time: to estimate the divergence time between mudskippers and other teleosts, as well as among the four mudskipper species, MCMCTree ( http://abacus.gene.ucl.ac.uk/software/paml.html ) from the PAML package [52] was used on 4D genes of each species and phylogenetic tree (mentioned in Supplementary Note 5 Phylogenetic tree construction) together with the molecular clock model. We set several reference divergence times (marked by red dots in several branches) from TimeTree database [53] ( http://www.timetree.org/ ) to calibrate the divergence times of other nodes. Detection of positively selected genes We extracted a total of 4,844 one-to-one orthologous gene families from seven teleosts (fugu, greenpuffer, stickleback, medaka, zebrafish, BP and PM) to identify PSGs. We generated multiple-protein alignments using MUSCLE version 3.8.31 (ref. 50 ) and trimAL version 1.4 (ref. 54 ) to remove gaps. These high-quality alignments were used to estimate three types of ω (the ratio of the rate of non-synonymous substitutions to the rate of synonymous substitutions) using two models of PAML [52] underlying species tree of these seven teleosts. In detail, branch model [55] (model=2, NSsites=0) was used to detect ω of appointed branch to test ( ω 0) and average ω of all the other branches ( ω 1) and basic model (model=0, NSsites=0) was used to estimate average of whole branches ( ω 2) and Orthologs with dS (the rate of synonymous substitution) >3 or ω 0>5 were removed [56] . Then χ 2 -test was used to check whether ω 2 was significantly higher than ω 1 and ω 0 with threshold P value<0.05, which hinted that these genes could be under positive selection or fast evolution. How to cite this article: You, X. et al. Mudskipper genomes provide insights into the terrestrial adaptation of amphibious fishes. Nat. Commun. 5:5594 doi: 10.1038/ncomms6594 (2014). Accession codes: Whole genome assemblies of the four mudskippers have been deposited in GenBank/EMBL/DDBJ under the accession codes JACK00000000 (BP), JACL00000000 (PM), JACM00000000 (PS) and JACN00000000 (SH).